Efficient preparation of unsymmetrical disulfides by nickel-catalyzed reductive coupling strategy Disulfides are widely found in natural products and find a wide range of applications in life sciences, materials chemistry and other fields. The preparation of disulfides mainly rely on oxidative couplings of two sulfur containing compounds. This strategy has many side reactions and other shortcomings. Herein, we describe the reductive nickel-catalyzed cross-electrophile coupling of unactivated alkyl bromides with symmetrical alkyl- and aryltetrasulfides to form alkyl-alkyl and aryl-alkyl unsymmetrical disulfides. This approach for disulfide synthesis is practical, relies on easily available, unfunctionalized substrates, and is scalable. We investigated the mechanism of this transformation and found that the tetrasulfide compound does not selectively break the central S–S bond, but regio-selectively generates trisulfide intermediates. Disulfides are widely found in natural products and have a wide range of applications in many fields, such as life science [1] , [2] , [3] and medical chemistry [4] , [5] . In the formation of protein tertiary structure, disulfide bonds play a central role [2] , [6] , [7] . The activity of many natural products and drugs depends on the exchange reaction of disulfide bonds in proteins [4] , [8] , [9] . The lipoic acid present in the mitochondria can increase the synthesis of ATP in the cell energy cycle [10] . Kottamide E has a five-membered ring disulfide structure, which has good anti-tumor and anti-inflammatory effects [11] . As a consequence, the efficient preparation of various functionalized disulfides is of continued interest (Fig. 1 ). Fig. 1: Representative biorelevant disulfide compounds. The importance of disulfides in life science, natural products, and other fields. Full size image Given the importance and predominance of disulfides in pharmaceuticals and bioactive compounds, chemists are continually seeking for efficient preparation strategies for multifunctional disulfides. While the preparation of symmetrical disulfide has been greatly developed [12] . Due to the limitation of the substrate structures, the preparation of unsymmetrical disulfide is still challenging. The traditional method for the construction of unsymmetrical disulfide compounds based on oxidative coupling of two different thiols (Fig. 2a ) [13] , [14] , [15] , [16] , [17] . In view of low yields, poor selectivities, and poor substrate universality, the development of a more efficient method for preparing unsymmetrical disulfide is desirable. In recent years, chemists have designed and synthesized many prefunctionalized/activated disulfurating reagents, and successfully constructed a series of functionalized unsymmetrical disulfides. Xian [18] , Xu [19] , and Wang [20] have independently disclosed their own disulfide reagents. In this field, Jiang’s group has made excellent achievement, by the introduction of the Mask group into the disulfide reagent, designed and synthesized a series of nucleophilic or electrophilic disulfide reagents, and efficiently constructed a series of highly functionalized polysulfide compounds (Fig. 2b ) [21] , [22] . On the basis of these studies, they designed and synthesized a series of new bilateral disulfurating reagents, which greatly expanded the construction of unsymmetrical disulfide compounds [23] , [24] . In 2020, the Pratt group demonstrated that tetrasulfides undergo efficient homolytic substitution with alkyl radicals, enabling the synthesis of a broad range of unsymmetrical disulfides (Fig. 2c ) [25] , [26] , [27] . This protocol showed mild reaction conditions and a large substrate scope. Fig. 2: Strategies for unsymmetrical disulfide assembly. a Traditional disulfuration by S–S bond formation. b Direct disulfuration via masked strategy. c Radical substitution on tetrasulfides. d Nickel-catalyzed reductive thiolation on tetrasulfides. Full size image Reductive coupling reactions of electrophiles avoid the preparation and use of organometallic reagents, have excellent compatibility with various functional groups, and provide an important method for the construction of C–C bonds [28] . In recent years, breakthroughs have been made in the research of this strategy, and a series of cross-coupling reactions involving C(sp 2 )-X and C(sp 3 )-X electrophiles have been realized [29] , [30] , [31] , [32] . In recent years, our group has used thiosulfonate as a sulfur source and constructed a series of highly functionalized sulfides and selenides under nickel-catalyzed reductive coupling conditions [33] , [34] , [35] . Inspired by Pratt’s work and combined with our previous work on reductive coupling reactions to synthesize sulfides, we reasoned that we can prepare unsymmetrical disulfides from alkyl halides through Nickel-catalyzed cross-electrophile coupling with tetrasulfide. Herein, we report on the successful development of a cross-coupling reaction of unactivated alkyl bromides with symmetrical tetrasulfides utilizing nickel-catalyzed reductive coupling strategy to construct unsymmetrical alkyl–alkyl disulfides and alkyl–aryl disulfides (Fig. 2d ). Reaction conditions survey Initially, we tried the reaction of 1-bromo-3-phenylpropane ( 1b ) with 1,4-di- tert -butyltetrasulfane ( 2a ), Ni(PPh 3 ) 2 Cl 2 (5 mol%), Mn (1.5 equiv), ligand (10 mol%) in (dry) DMF at 40 °C for 12 h under N 2 atmosphere. Gratifyingly, the reaction proceeded smoothly to give a mixture products of 1-( tert -butyl)-2-(3-phenylpropyl)disulfane ( 3b ) and 1-( tert -butyl)-3-(3-phenylpropyl)trisulfane ( 3b ′) (2.8:1) (However, the disulfide could not be separated from the trisulfide). Surprisingly, when we extended the reaction time to 24 h, the ratio of 3b and 3b ′ increased to 31:1. With this promising results in hand, we tried to further optimize the reaction conditions (see Supplementary Tables 1 – 3 for more details). 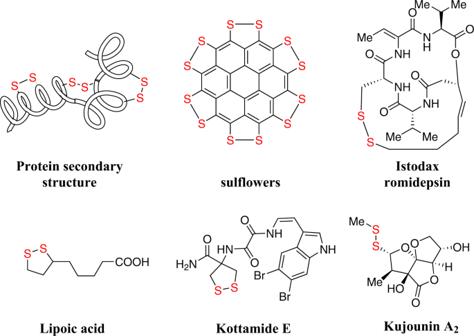Fig. 1: Representative biorelevant disulfide compounds. The importance of disulfides in life science, natural products, and other fields. As briefly illustrated in Table 1 , after systematic exploring the reductive coupling with L1 as the ligand, Ni(acac) 2 was chosen as catalyst as its use lead to the highest yield and selectivity (Table 1 , entries 1–5). Next, we conducted the ligand optimization with a series of bipyridine ligands and phenanthroline ligands. As a result, L1 provided superior result (Table 1 , entries 6–12). Then, we tried the reactions in several different solvents, such as DMF, DMA, DMSO, and MeCN. It was found that DMF was crucial for the successful transformation of 1b (Table 1 , entries 13–15). When Zn was used instead of Mn, the target product 3b could not be obtained (Table 1 , entry 16). Table 1 Optimization of the reaction conditions a,b . Full size table Generality of protocol With the optimized reaction conditions in hand, we set out to assess the generality of this protocol (Fig. 3 ). Hence, primary alkyl bromides bearing various functional groups were employed in the reactions with 1,4-di- tert -butyltetrasulfane 2a . To our delight, the length of the carbon chain had no effect on the reaction, the desired disulfide products 3a – 3f could be obtained in good to excellent yields. The reaction of 3-(2-bromoethyl)-1 H -indole 1g with 1,4-di- tert -butyltetrasulfane ( 2a ) gave the target product 3g in excellent yield. Satisfactorily, a wide range of substituents, including alcohol, siloxane, phosphonate were well-tolerated under this mild reaction condition. The target products 3h – 3j were isolated in medium to good yields. However, the reaction of ethyl 6-bromohexanoate 1k with 1,4-di- tert -butyltetrasulfane ( 2a ) gave the target product 3k in only 34% yield. It should be noted that the reaction of methyl( R )-3-bromo-2-(( tert -butoxycarbonyl)amino)propanoate ( 1l ) with 1,4-di- tert -butyltetrasulfane ( 2a ) furnished the desired product 3l in 82% yield. This greatly expanded the application of this strategy in the construction of unsymmetrical disulfide compounds. Surprisingly, the reaction of 1-bromo-6-chlorohexane ( 1m ) with tetrasulfane 2a not only could delivered the expected product 3m in 67% yield, but also led to 3m ′ in 20% yield. This demonstrated that this strategy is also applicable to alkyl chlorides. When tert -butyl (3-bromopropyl)carbamate ( 1n ), 2-(3-bromopropyl)isoindoline-1,3-dione ( 1o ) and 4-bromobutanenitrile ( 1p) were applied to the reaction respectively, a mixture of trisulfide compounds and disulfides were obtained ( 3n – 3p , 3n ′– 3p ′). In contrast, the reaction of secondary bromide, tertiary bromide and dibromide failed to give the desired products. According to the related works of Prof. Gong [36] , [37] , [38] , we speculate that the possible reason is that the oxidative addition of nickel(0) and tetrasulfide furnishes nickel(II) intermediate, this intermediate is very sterically hindered due to the coordination of the ligand. Therefore, when secondary bromine and tertiary bromine participate in the reaction, the target products could not be obtained due to the steric hindrance effect. Fig. 3: Scope of primary alkyl bromides. a Reaction conditions: primary alkyl bromides 1 (0.20 mmol, 1.0 equiv. ), 2a (0.24 mmol, 1.2 equiv. ), Ni(acac) 2 (5.0 mol%); L1 (10 mol%), Mn (0.30 mmol, 1.5 equiv. ), DMF (1 mL), N 2 atmosphere, 40 °C, 24 h. b Isolated yield. c 80 °C. Full size image Encouraged by the above achievements, we turned our attention to exploring other symmetrical tetrasulfide compounds (Fig. 4 ). However, under the previously optimized conditions, only 1,4-dibenzyltetrasulfane and 1,4-dicyclohexyltetrasulfane gave the target products 4a and 4b with a high selectivity. When other tetrasulfides were applied to the reaction, a mixture products of trisulfide and tetrasulfide was obtained. Therefore, we adjusted the reaction conditions (see Supplementary Tables 4 – 6 for more details). Next, we reexamined the activity of various symmetric tetrasulfide substrates. It is exciting that regardless of whether it is branched liner tetrasulfides, the desired products could be obtained with high chemoselectivity ( 4c – 4e ). The reaction of 1-(2-bromoethyl)-4-methoxybenzene with 1,2-bis(furan-2-ylmethyl)disulfane gave the desired product 4f in moderate yield. However, when 1,4-diisopropyltetrasulfane and 1,4-di- p -tolyltetrasulfane were applied to the reaction, respectively, a mixture product of trisulfide and disulfide were formed ( 4g – 4h , 4g ′– 4h ′). To demonstrate the synthetic value of our method, we explored the scale-up with (3-bromopropyl)benzene ( 1b ) and 1,4-di -tert -butyltetrasulfane ( 2a ) under the otherwise identical reaction conditions. To our delight, the desired product 3b could be obtained in 90% yield. Fig. 4: Scope of tetrasulfides 2. Reaction conditions: Primary alkyl bromides 1 (0.20 mmol, 1.0 equiv. 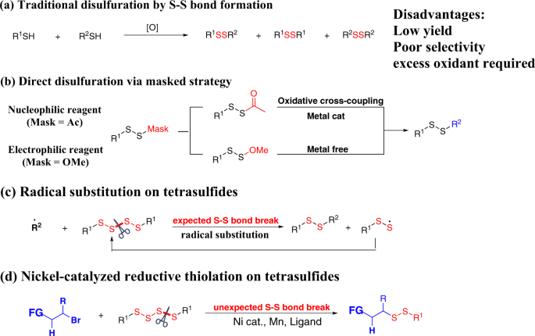Fig. 2: Strategies for unsymmetrical disulfide assembly. aTraditional disulfuration by S–S bond formation.bDirect disulfuration via masked strategy.cRadical substitution on tetrasulfides.dNickel-catalyzed reductive thiolation on tetrasulfides. ), symmetrical tetrasulfides 2 (0.24 mmol, 1.2 equiv. ), Mn (0.30 mmol, 1.5 equiv. ), DMF (1 mL), N 2 atmosphere. a Ni(acac) 2 (5.0 mol%), L1 (10 mol%); 40 °C, 24 h. b NiF 2 (5.0 mol%), L2 (10 mol%), 80 °C; 24 h. c Isolated yield. Full size image Mechanistic studies Subsequently, mechanistic studies were conducted to gain insights into the reaction pathway (see Supplementary Figs. 1 – 3 for more details). When Ni(PPh 3 ) 2 Cl 2 was applied as the catalyst, the reaction proceeded to give a mixture products of 3b and 3b ′ (2.8:1) (Fig. 5a ). 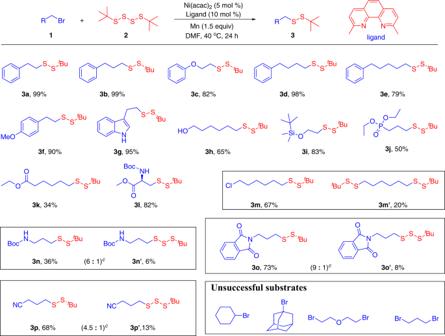Fig. 3: Scope of primary alkyl bromides. aReaction conditions: primary alkyl bromides1(0.20 mmol, 1.0 equiv.),2a(0.24 mmol, 1.2 equiv.), Ni(acac)2(5.0 mol%); L1 (10 mol%), Mn (0.30 mmol, 1.5 equiv.), DMF (1 mL), N2atmosphere, 40 °C, 24 h.bIsolated yield.c80 °C. Surprisingly, when we extended the reaction time to 24 h, the ratio of 3b and 3b ′ changed 31:1 (Fig. 5b ). This indicated that product 3b ′ might be a reaction intermediate. Therefore, we prepared the trisulfide product 2i , regrettably, the reaction of (3-bromopropyl)benzene ( 1b ) with 1,3-dibenzyltrisulfane ( 2i ) did not give the target product 7 , but the trisulfide product 3i itself was converted into disulfide compound 2j ( 2i : 2j = 1:13) (Fig. 5c ). This finding indicated that trisulfide is more likely to transform into disulfide. Fig. 5: Key mechanistic findings. a The reaction of 1b and 2a under standard conditions for 12 h. b The reaction of 1b and 2a under standard conditions for 24 h. c The reaction of 1b and 2j under standard conditions for 24 h. d The catalytic system was analyzed by high-resolution mass spectrometry. e Investigation on the reaction mode of trisulfide 6a under different conditions. f Investigation on the reaction mode of unsymmetrical trisulfide 8 under different conditions. g The reaction of 1,2-dibenzyldisulfane 7a and 1,2-di-tert-butyldisulfane 9 under standard conditions for 24 h. Full size image Next, we performed high-resolution mass spectrometry to analyse the catalytic system. 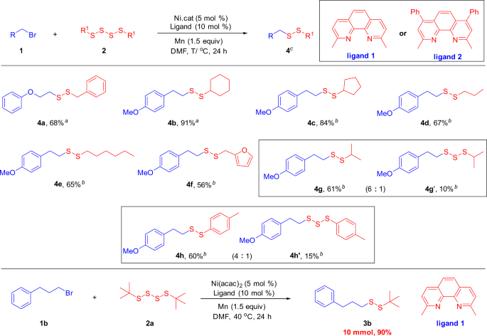Fig. 4: Scope of tetrasulfides 2. Reaction conditions: Primary alkyl bromides1(0.20 mmol, 1.0 equiv.), symmetrical tetrasulfides2(0.24 mmol, 1.2 equiv.), Mn (0.30 mmol, 1.5 equiv.), DMF (1 mL), N2atmosphere.aNi(acac)2(5.0 mol%),L1(10 mol%); 40 °C, 24 h.bNiF2(5.0 mol%),L2(10 mol%), 80 °C; 24 h.cIsolated yield. 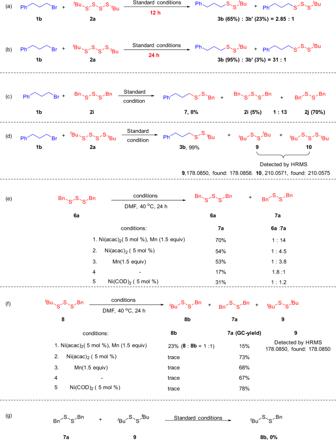Fig. 5: Key mechanistic findings. aThe reaction of1band2aunder standard conditions for 12 h.bThe reaction of1band2aunder standard conditions for 24 h.cThe reaction of1band2junder standard conditions for 24 h.dThe catalytic system was analyzed by high-resolution mass spectrometry.eInvestigation on the reaction mode of trisulfide6aunder different conditions.fInvestigation on the reaction mode of unsymmetrical trisulfide8under different conditions.gThe reaction of 1,2-dibenzyldisulfane7aand 1,2-di-tert-butyldisulfane9under standard conditions for 24 h. 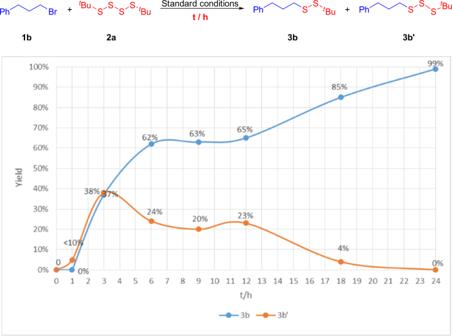Fig. 6: Investigation of the reaction process. The investigation of the template reaction under standard conditions at different time by GC-Ms. Under the standard conditions, only trace amount of the disulfide product 9 and the trisulfide product 10 were detected by careful HRMS analysis (Fig. 5d ). We likewise investigated the viability for a conversion of trisulfides to disulfides (Fig. 5e ) (see Supplementary Figs. 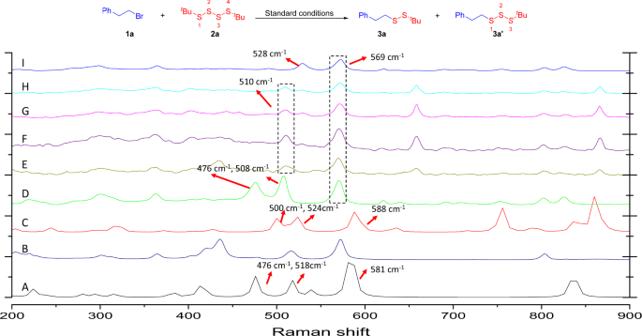Fig. 7: Raman study (I). Raman caculation spectra of (A)2acalculated data. (B)2a. (C)3a′ calculated data. (D)3a′. (E)1awith2aunder optimized reaction conditions,t= 1 h, (F)1awith2aunder optimized reaction conditions,t= 4 h, (G)1awith2aunder optimized reaction conditions,t= 8 h, (H)1bwith2aunder optimized reaction conditions,t= 1 h. (I)3a. 4 , 5 and Table 7 for more details). Through detailed experimentation, it was demonstrated that both the nickel catalyst and the manganese play a crucial role in the conversion of trisulfides to disulfides. According to a previous study [19] , we furthermore prepared unsymmetric trisulfide 8 . Under standard conditions, 1-benzyl-2-(tert-butyl)disulfane 8b and 1,2-dibenzyldisulfane 7a could be obtained in 23% and 15% yields, respectively (with a conversion of 8 being 77%). Only trace amounts of the disulfide product 9 was detected by HRMS analysis. We investigated the conditions for the conversion of trisulfide 8 to disulfide 8b . It was found that when the reaction conditions were modified, only trace amounts of unsymmetric disulfide 8b and symmetric disulfide 9 were detected and 7a was formed as the main product (Fig. 5f ). We further investigated the cross reaction of 1,2-dibenzyldisulfane 7a and 1,2-di- tert -butyldisulfane 9 under otherwise identical reaction conditions, which notably failed to give unsymmetrical disulfide 8b . This result provides strong support against an initial formation of two symmetrical disulfides from the trisulfide. Therefore, a subsequent cross reaction to form the unsymmetric disulfide is unlikely to be operative (Fig. 5g ). Subsequently, we investigated the standard reaction at different reaction times (Fig. 6 ). Through detailed GC-MS analysis, we found that when the reaction proceeded for 1 h, 3b could not be detected, while instead only the trisulfide product 3b ′ was detected. When the reaction time was prolonged to 3 h, the ratio of products 3b and 3b ′ was close to 1:1. Thereafter, the yield of 3b′ gradually decreased. These experimental findings render the possibility of nickel inserting into the central S–S bond of the tetrasulfide unlikely. Instead our observations provide further strong support for trisulfide serving as the key intermediate. Fig. 6: Investigation of the reaction process. The investigation of the template reaction under standard conditions at different time by GC-Ms. Full size image There is increasing literature precedence for S–S bonds in polysulfides serving as strong Raman scatterers [39] . Thus, we exploited the enormous enhancement in the Raman intensity of polysulfides in order to understand the working mode of our reductive coupling. To aid the assignment, Raman frequency calculations for 2a (Fig. 7 , A), 3a (Fig. 7 , I), and 3a ′ (Fig. 7 , C) were carried out at the UB3LYP/aug-cc-pV(Q + d)Z-DK level. Thus, Raman frequency calculations for 2a featured peaks at 476 cm −1 , 518 cm −1 , and 581 cm −1 corresponding to the S(2)–S(3), S(1)–S(2), and ( t Bu)C-S stretching of tetrasulfide, respectively. As Raman frequency calculations for 3a ′, peaks at 500 cm −1 , 524 cm −1 , and 588 cm −1 correspond to the S(1)–S(2), S(2)–S(3), and ( t Bu)C-S stretching of trisulfide 3a ′, respectively. As Raman frequency for 3a ′, peaks at 476 cm −1 , 508 cm −1 , and 569 cm −1 correspond to the S(1)–S(2), S(2)–S(3), and ( t Bu)C-S stretching of trisulfide 3a ′, respectively. This result is most likely match with the calculated data with −24 cm −1 relative error. As Raman frequency for 3a , peaks at 528 cm −1 , and 569 cm −1 correspond to the S–S, and C-S stretching of disulfide 3a , respectively. We further monitored the reaction of 1a and 2a under the standard reaction conditions with the Raman spectroscopy (Fig. 7 , E–H). It was found that 476 cm −1 correspond to the S(2)–S(3) of tetrasulfide 2a decreased and a significant increase in 528 cm −1 peak ( ν 1 ), which is the characteristic S–S stretching of 3a . We also investigated the Raman spectroscopy of 3a ′ under the standard reaction conditions (Fig. 8 , C–F). It was found that peak at 476 cm −1 and 508 cm −1 corresponds to the S(1)–S(2) and S(2)–S(3) of trisulfide 3a ′ decreased dramatically. This result means that S–S–S bond of trisulfide 3a ′ could be quickly activated under the reaction conditions. Fig. 7: Raman study (I). Raman caculation spectra of (A) 2a calculated data. (B) 2a . (C) 3a ′ calculated data. (D) 3a ′. (E) 1a with 2a under optimized reaction conditions, t = 1 h, (F) 1a with 2a under optimized reaction conditions, t = 4 h, (G) 1a with 2a under optimized reaction conditions, t = 8 h, (H) 1b with 2a under optimized reaction conditions, t = 1 h. (I) 3a . Full size image Fig. 8: Raman study (II). Raman spectra of (A) 3a ′ calculated data, (B) 3a ′. (C) 3a ′ under optimized reaction conditions, t = 1 h, (D) 3a ′ under optimized reaction conditions, t = 4 h, (E) 3a ′ under optimized reaction conditions, t = 8 h, (F) 3a ′ under optimized reaction conditions, t = 12 h, (G) 3a . Full size image Based on our detailed experimental and computational findings and the literature reports [33] , [34] , [35] , [40] , [41] , [42] , we propose a plausible reaction mechanism in Fig. 9 . The in situ reduction of nickel(II) by manganese affords Ni(0)(L) 2 I . The tetrasulfide 2 could be activated by Ni(0) or Mn. The oxidative addition of I and tetrasulfide 2 in the presence of Ni(0) or Mn furnishes intermediate II , which reacts with an alkyl radical to form nickel(III)(L) intermediate III . The reductive elimination of III leads to trisulfide intermediate IV and the nickel(I)(L) 2 species V . Next, the nickel(I) V reacts with alkyl bromide 1 to give the alkyl radical and nickel(II)(L) VI . Finally, the reduction of intermediate VI regenerates complex I and disulfide by-product. On the other hand, the oxidative addition of I and trisulfide IV in the presence of Ni(0) affords intermediate VII (both intermediates VII-1 and intermediate VII-2 are possible). VII is converted into intermediate VIII with releasing polysulfur anion and S 8 (polysulfur anion and S 8 were confirmed by XRD. For details, please see Supplementary Fig. 5 ). The reductive elimination of VIII furnish disulfide and complex I . Fig. 9: Plausible catalytic cycle. Possible reaction mechanism for nickel-catalyzed reduction of disulfide. Full size image In conclusion, we have reported on a nickel-catalyzed reductive disulfideization of unactivated alkyl bromides with organic tetrasulfides. The reaction proceeded with excellent chemoselectivity under mild conditions, and enabled the efficient assembly of diversely decorated disulfides. Detailed mechanistic studies revealed that, in contrast to literature precedence, the tetrasulfide compound did not undergo scission of the central S–S bond, but selectively formed substituted trisulfides as key intermediates. General procedures Synthesis of 3b In a glovebox, an oven-dried screw-capped 8 mL vial equipped with a magnetic stir bar was charged with (3-bromopropyl)benzene ( 1b , 39.6 mg, 0.2 mmol) and 1,4-di- tert -butyltetrasulfane ( 2a , 58.1 mg 0.24 mmol), Ni(acac) 2 (2.6 mg, 5.0 mol%), L1 (10 mol%), Mn (1.5 equiv), DMF (1.0 mL) was added via syringe. The reaction mixture was stirred for 24 h at 40 °C. After 24 h, the crude reaction mixture was diluted with ethyl acetate (20 mL) and washed with water (20 mL × 3). 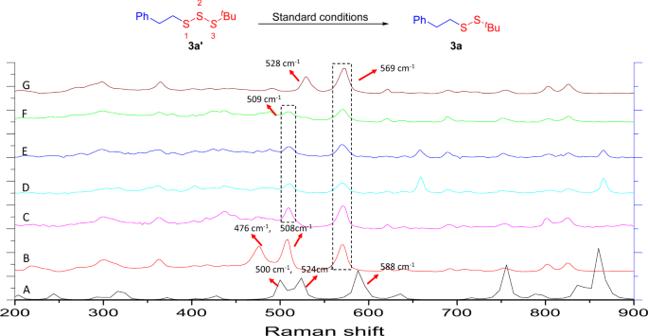Fig. 8: Raman study (II). Raman spectra of (A)3a′ calculated data, (B)3a′. (C)3a′ under optimized reaction conditions,t= 1 h, (D)3a′ under optimized reaction conditions,t= 4 h, (E)3a′ under optimized reaction conditions,t= 8 h, (F)3a′ under optimized reaction conditions,t= 12 h, (G)3a. 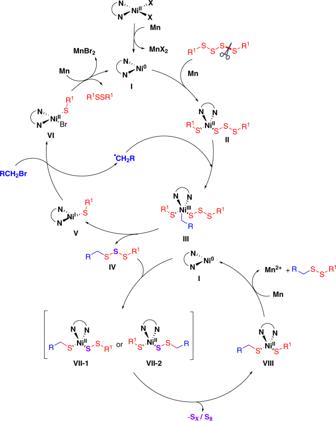Fig. 9: Plausible catalytic cycle. Possible reaction mechanism for nickel-catalyzed reduction of disulfide. The organic layer was dried over Na 2 SO 4 , filtered, and concentrated. The residue was purified by flash chromatography to afford pure product 3b (99% yield). Synthesis of 4h In a glovebox, an oven-dried screw-capped 8 mL vial equipped with a magnetic stir bar was charged with 1-(2-bromoethyl)-4-methoxybenzene ( 1f , 42.8 mg, 0.2 mmol) and 1,4-di- p -tolyltetrasulfane ( 2h , 74.4 mg 0.24 mmol), NiF 2 (1.0 mg, 5.0 mol%), L1 (10 mol%), Mn (1.5 equiv), DMF (1.0 mL) was added via syringe. The reaction mixture was stirred at 80 °C for 24 h. After 24 h, the crude reaction mixture was diluted with ethyl acetate (20 mL) and washed with water (20 mL × 3). The organic layer was dried over Na 2 SO 4 , filtered, and concentrated. The residue was purified by flash chromatography to afford products of 4h and 4h ′.